High-power biofuel cell textiles from woven biscrolled carbon nanotube yarns Biofuel cells that generate electricity from glucose in blood are promising for powering implantable biomedical devices. Immobilizing interconnected enzyme and redox mediator in a highly conducting, porous electrode maximizes their interaction with the electrolyte and minimizes diffusion distances for fuel and oxidant, thereby enhancing power density. Here we report that our separator-free carbon nanotube yarn biofuel cells provide an open-circuit voltage of 0.70 V, and a maximum areal power density of 2.18 mW cm −2 that is three times higher than for previous carbon nanotube yarn biofuel cells. Biofuel cell operation in human serum provides high areal power output, as well as markedly increased lifetime (83% remained after 24 h), compared with previous unprotected biofuel cells. Our biscrolled yarn biofuel cells are woven into textiles having the mechanical robustness needed for implantation for glucose energy harvesting. Biofuel cells (BFCs) [1] , [2] are particularly interesting as power sources for implantable biomedical devices, such as cardiac pacemakers, nerve-stimulators and drug-delivering pumps [1] . Currently developed BFCs are typically limited by low power output and short lifetime. Improved performance has been achieved by increasing the loading of enzymes immobilized on carbon nanotube yarn electrodes [3] and carbon nanotube composite disk electrodes [4] . Redox mediators also enhance performance by facilitating electron transfer between the enzyme and the current collector [2] , [5] . The recently described biscrolling process [6] , [7] provides a promising method for fabricating multi-walled carbon nanotube (MWCNT) yarn electrodes that can be woven into BFC textiles. Biscrolling involves coating a MWCNT sheet host with a guest material and subsequent twist-spinning of the host–guest stack to produce a yarn that can contain over 95 wt% of guest. The high electrical conductivity, mechanical strength and flexibility of the hybrid yarns, combined with the compressive pressure generated by twist insertion, provide excellent electrical connection between guests and hosts for charge collection, while providing the mechanical robustness needed for weaving, sewing, knotting and braiding [7] . The main challenge in developing BFC electrodes using the biscrolling method is the immobilization of hydrophilic enzymes, cross-linker and redox mediator guests within the hydrophobic MWCNT host. MWCNT sheets cannot be wetted by surfactant-free aqueous solutions unless the nanotube surfaces are modified by charge injection or surface derivatization [8] . In addition, unsupported MWCNT sheets irregularly collapse when contacted with liquids and dried, which restricts the original biscrolling process to deposition of dry powders or complicated processing. For example, filtration-based deposition of liquid-dispersed powder on a nanotube sheet ribbon and subsequent immersion of the filter-paper-supported host/guest stack into a liquid bath that dissolved the filter paper, enable subsequent twist insertion into the host/guest ribbon stack while it is in the liquid bath [7] . Here we overcome these processing problems by first stabilizing the carbon MWCNT sheets structure by using vapour-phase polymerization to coat poly(3,4-ethylenedioxythiophene), PEDOT [9] , on the individual MWCNT bundles. The coated MWCNTs are then hydrophilic, and the MWCNT sheet network increases mechanical strength and electrical connectivity [9] . The hydrophilic PEDOT coating enables high loading of enzyme and redox mediator, which are deposed together with a cross-linker in a one-step process from aqueous solution. Biscrolling this assembly produces a yarn that is highly flexible and easily woven as electrodes into a BFC textile. This novel strategy builds upon previous success in using PEDOT for planar electrode-based BFCs [10] , [11] . Structure of biscrolled BFC yarn electrodes Scanning electron microscopy images show that the guest-free PEDOT/MWCNT sheet ( Supplementary Fig. 1 ) and the biscrolled yarn electrodes filled with guest ( Fig. 1b,c ) have highly oriented, and porous structures. Cross-sectional images of the biscrolled yarn cathode ( Fig. 1d,e ) and anode show vascular-like corridors formed from scrolled PEDOT/MWCNT sheets, which trap the guests within the yarn such that structures likely allow fast mass transport of glucose and oxygen for oxidation and reduction within the yarn electrodes. Non-modified guest-free PEDOT/MWCNT yarn was conducting (40.0 S cm −1 ) and mechanically strong (72±9.2 MPa), and its tensile strain was 10±2.4%. Despite the presence of 88±0.6 and 81±0.9 wt% of yarn guest for anode and cathode yarns, respectively, the anode and cathode yarns also retained high strength (71±11.2 and 139±8.6 MPa, respectively) ( Supplementary Fig. 2 ) and conductivity (19.2 and 14.7 S cm −1 , respectively). 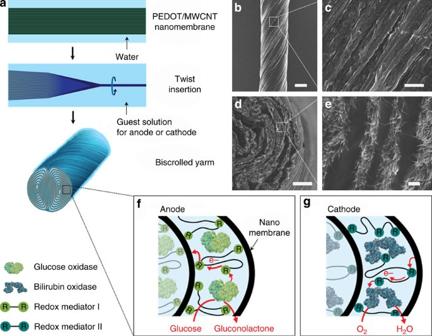Figure 1: The fabrication and structure of biscrolled yarn electrodes for BFCs. (a) Schematic illustration of the fabrication method for biscrolled yarn electrodes. (b,c) SEM micrographs showing the surface of a 50-μm diameter biscrolled yarn cathode based on PEDOT/MWCNT host. The scale bars were 20 μm and 500 nm, respectively. The yarn bias angle (the angle between the MWCNT fibre direction on the yarn surface and the yarn direction) is ~37°. (d,e) SEM cross-section images at low and high magnifications of the fracture surface of a biscrolled yarn cathode, which shows yarn corridors between scrolled PEDOT/MWCNT sheets that contain the yarn guests. The scale bars were 5 μm and 500 nm, respectively. (f) Schematic illustration of the structure and function of BFC anode yarns, which indicate associated electron transfer processes and chemical transformations. The enzyme and redox mediator polymer used were glucose oxidase (GOx) and mediator I. (g) The structure and function of BFC cathode yarns. The enzyme and redox mediator polymer used were bilirubin oxidase (BOD) and mediator II. Figure 1: The fabrication and structure of biscrolled yarn electrodes for BFCs. ( a ) Schematic illustration of the fabrication method for biscrolled yarn electrodes. ( b , c ) SEM micrographs showing the surface of a 50-μm diameter biscrolled yarn cathode based on PEDOT/MWCNT host. The scale bars were 20 μm and 500 nm, respectively. The yarn bias angle (the angle between the MWCNT fibre direction on the yarn surface and the yarn direction) is ~37°. ( d , e ) SEM cross-section images at low and high magnifications of the fracture surface of a biscrolled yarn cathode, which shows yarn corridors between scrolled PEDOT/MWCNT sheets that contain the yarn guests. The scale bars were 5 μm and 500 nm, respectively. ( f ) Schematic illustration of the structure and function of BFC anode yarns, which indicate associated electron transfer processes and chemical transformations. The enzyme and redox mediator polymer used were glucose oxidase (GOx) and mediator I. ( g ) The structure and function of BFC cathode yarns. The enzyme and redox mediator polymer used were bilirubin oxidase (BOD) and mediator II. Full size image Choice of different enzymes and redox mediators for the opposite electrodes determines where oxidation and reduction occurs, thereby eliminating the need for a separator giving a simple, single-compartment BFC, which helps enable high current densities. Osmium-containing conducting polymers [12] were chosen as redox mediators to facilitate rapid electron transfer between the enzymes and the scrolled PEDOT-coated MWCNT sheets. Simply inserting twists into free-standing MWCNT sheet, which supported an enzyme, enzyme cross-linker and redox mediator, conveniently produced a biscrolled yarn in which these guests were integrated in nanoscale proximity to the host MWCNT/PEDOT current collector ( Fig. 1 ). The enzyme and redox polymer used were glucose oxidase (GOx) and poly( N -vinylimidazole)-[Os(4,4′-dimethoxy-2,2′-bipyridine) 2 Cl]) +/2+ (redox mediator I) for anode ( Fig. 1f ) and bilirubin oxidase (BOD) and poly(acryl amide)-poly( N -vinylimidazole)-[Os(4,4′-dichloro-2,2′-bipyridine) 2 ]) +/2+ (redox mediator II) for cathode ( Fig. 1g ). Each enzyme was cross-linked by poly(ethylene glycol) diglycidyl ether (PEGDGE). Performance of biscrolled yarn BFC anode and cathode Anodic and cathodic performances were optimized by adjusting the weight percentages of the enzymes in the enzyme/redox mediator solution used for coating the PEDOT/MWCNT sheets before biscrolling. The fuel cell electrolyte was 20 mmol l −1 phosphate-buffered 0.14 mol l −1 NaCl solution (PBS). Especially for the cathode, it was observed that the current density strongly depended on the weight percentage of enzyme in the coating solution ( Fig. 2 ), reaching a maximum current density at about 41 wt% BOD. Above 45 wt% of BOD, the current density rapidly declined probably as a result of precipitation observed in the guest solution, which reduced the amount of guest incorporated during biscrolling and/or reduced their activity in the bioscrolled yarn due to aggregation or reduced yarn porosity. Since ~41 wt% enzyme optimized performance for both anode and cathode, this concentration was used for both electrodes. The fabricated electrodes were characterized by cyclic voltammetry under argon and the observed oxidation and reduction peaks confirm the immobilization of the redox polymer guest on the electrode surface (insets of Fig. 3b,c ). 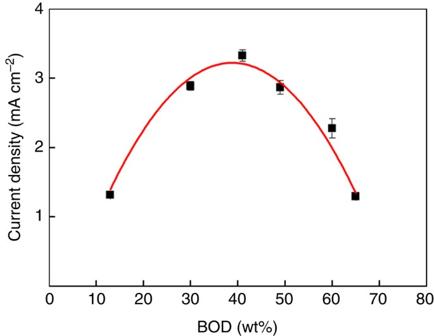Figure 2: The dependence of areal current density on the enzyme concentration. These data were obtained by linear sweep voltammetry for a biscrolled cathode yarn that contains bilirubin oxidase (BOD) as the enzyme. The error bars show the s.d. of maximum areal current density for three cases. Figure 2: The dependence of areal current density on the enzyme concentration. These data were obtained by linear sweep voltammetry for a biscrolled cathode yarn that contains bilirubin oxidase (BOD) as the enzyme. The error bars show the s.d. of maximum areal current density for three cases. 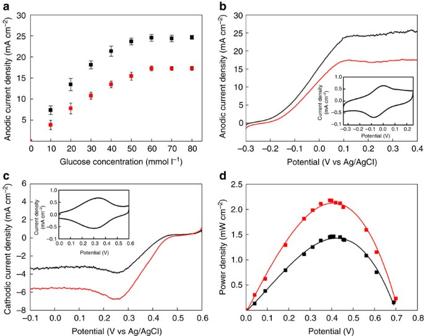Figure 3: Performance of the biscrolled BFC yarn electrodes and the complete BFC. (a) Areal current density for the BFC yarn anode as a function of glucose concentration. The error bars show the s.d. from the mean value of current densities for three independent experiments. (b) Polarization curves for the BFC yarn anode at 60 mmol l−1glucose concentration. Inset: cyclic voltammetry curve showing the peak of redox polymer I for anode under argon. (c) Polarization curve for the BFC yarn cathode at 60 mmol l−1glucose concentration. Inset: cyclic voltammetry showing the peak of redox polymer II for cathode under argon. (d) Areal power density as a function of potential for the complete BFC system at 60 mmol l−1glucose concentration. The experiment was carried out under 20 mmol l−1phosphate-buffered saline solution (temperature: 37 °C, scan rate: 5 mV s−1), when saturated with air (black symbols and curves) and O2(red symbols and curves). Full size image Figure 3: Performance of the biscrolled BFC yarn electrodes and the complete BFC. ( a ) Areal current density for the BFC yarn anode as a function of glucose concentration. The error bars show the s.d. from the mean value of current densities for three independent experiments. ( b ) Polarization curves for the BFC yarn anode at 60 mmol l −1 glucose concentration. Inset: cyclic voltammetry curve showing the peak of redox polymer I for anode under argon. ( c ) Polarization curve for the BFC yarn cathode at 60 mmol l −1 glucose concentration. Inset: cyclic voltammetry showing the peak of redox polymer II for cathode under argon. ( d ) Areal power density as a function of potential for the complete BFC system at 60 mmol l −1 glucose concentration. The experiment was carried out under 20 mmol l −1 phosphate-buffered saline solution (temperature: 37 °C, scan rate: 5 mV s −1 ), when saturated with air (black symbols and curves) and O 2 (red symbols and curves). Full size image Increasing the concentration of the glucose fuel from 0 to 60 mmol l −1 increased the anodic current up to 24.7 mA cm −2 for operation in air-saturated electrolyte, as shown in Fig. 3a . For glucose concentrations above 60 mmol l −1 the current density was unchanged, due to the Michaelis–Menten type behaviour [12] of the GOx enzyme. For operation using oxygen-saturated electrolyte, the maximum anode current decreased to 17.2 mA cm −2 as a result of a competing GOx-catalysed side reaction, generating hydrogen peroxide from O 2 and less efficient electron transfer. The competition effect is more pronounced at low glucose concentrations where the current density in O 2 is only 50% of that in air, whereas this fraction increases to 70% at higher glucose levels. On the other hand, cathodic performance ( Fig. 3c ) reached a plateau current density of 3.3 mA cm −2 for air-saturated electrolyte compared with 5.6 mA cm −2 for O 2 saturation. As observed previously, the cathodic current density does not increase in proportion to the oxygen concentration [13] . Our observed current densities are high, although the specific activity of the cathodic enzyme was relatively low compared with the specific activity of the purified BOD enzyme used for a BFC based on carbon single-wall nanotubes [3] . Performance of complete BFC in synthetic electrolyte A complete BFC having biscrolled anode and cathode yarns generated an open-circuit voltage of +0.70 V when operated in 60 mmol l −1 oxygenated buffer, which agrees with the difference in potentials for the onset of catalytic oxidation of glucose at the anode and catalytic oxygen reduction at the cathode (−0.30 V in Fig. 3b and 0.50 V versus Ag/AgCl in Fig. 3c , respectively). As shown in Fig. 3d , a maximum areal power density of 2.18 mW cm −2 (based on the external surface area of the yarn electrode and corresponding to a volumetric power density of 793 mW cm −3 , based on total electrode volume) was obtained at an operating voltage of 0.40 V when using the oxygen-saturated, 60 mmol l −1 glucose electrolyte, which reduced to 1.46 mW cm −2 for the equivalent air-saturated electrolyte and the same operating voltage. The maximum realized areal power density of the biscrolled yarn BFC compare favourably with previous CNT systems, although direct comparisons are difficult owing to different experimental conditions. The highest power density of the biscrolled yarn BFC (2.18 mW cm −2 ) in oxygen-saturated PBS buffer solution with 60 mmol l −1 glucose solution is three times that for BFC-exploiting solution-spun single-wall nanotube fibres (0.74 mW cm −2 ) [3] in air-saturated 15-mmol l −1 glucose buffer solution; nearly double that for a mediator-free BFC based on compressed MWCNT/enzyme disks (1.3 mW cm −2 ) [4] in air-saturated 5-mmol l −1 glucose buffer solution; and even higher than for a two-layer-stacked CNT-film-based flexible BFC (1.8 mW cm −2 ) [14] in oxygen-saturated 200 mmol l −1 fructose buffer solution. These areal power densities are normalized with respect to the surface area of an electrode, which is the same for both anode and cathode. Like for supercapacitors [15] , this areal power density is the specially important figure of merit for a BFC textile, since it determines the power output for given area textile, which could be conveniently scrolled into a compact cylinder through whose corridors the blood circulates. BFC performance and stability in human serum In human serum, anionic chemical species, such as urate, chloride ion and ascorbic acid, are known to decrease BFC activity within a few hours [16] , [17] , [18] . Consequently, we here characterize at 37 °C both fuel cell power output and the time dependence of this output for both human serum and in a reference PBS electrolyte containing 7 mmol l −1 glucose concentration, which is within the normal glucose concentration range of human blood. Cyclic voltammetry for anode and cathode electrodes in human serum condition were shown in the Supplementary Fig. 3 . 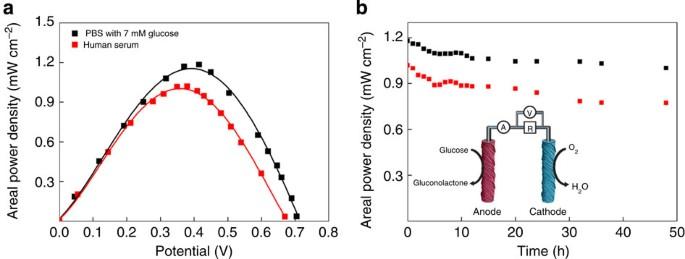Figure 4: Performance comparisons of BFCs in PBS and in human serum. (a) Areal power density as a function of cell voltage for a biscrolled yarn BFC in 7 mmol l−1glucose-concentrated PBS (filled black squares and curve) and in human serum (filled red squares and curve). (b) Dependence of areal power output on time for a biscrolled yarn BFC (poised at 0.40 V) in 7 mmol l−1glucose-concentrated PBS (filled black squares) and in human serum (filled red squares) at 37 °C. The inset illustrates the redox processes and indicates the resistance (R) of the applied external load and the location of voltage (V) and current (A) measuring devices. Figure 4a shows that comparable areal power densities versus cell potential are obtained using both human serum and the reference PBS electrolyte (after a pre-testing time for stabilizing the electrochemical reaction). The areal power density (1.02 mW cm −2 ) of our biscrolled yarn BFC in human serum is nearly as high at the 1.18 mW cm −2 obtained for the biscrolled BFC in PBS electrolyte containing 7 mmol l −1 glucose concentration. Figure 4: Performance comparisons of BFCs in PBS and in human serum. ( a ) Areal power density as a function of cell voltage for a biscrolled yarn BFC in 7 mmol l −1 glucose-concentrated PBS (filled black squares and curve) and in human serum (filled red squares and curve). ( b ) Dependence of areal power output on time for a biscrolled yarn BFC (poised at 0.40 V) in 7 mmol l −1 glucose-concentrated PBS (filled black squares) and in human serum (filled red squares) at 37 °C. The inset illustrates the redox processes and indicates the resistance (R) of the applied external load and the location of voltage (V) and current (A) measuring devices. Full size image Figure 4b shows that the power output (for cells poised at 0.40 V under air) is relatively stable and similar for yarn BFCs using either human serum or the PBS electrolyte (for the 12-h period when glucose concentration is not replenished and any added oxygen concentration depends on air contact with the stirred fuel cell electrolyte). This stability suggests that the structure of fuel cell yarn must be providing inherent stabilization. Such stabilization without the use of a protecting ionically conducting barrier (which can degrade power density performance) is important for possible future applications for harvesting energy in the human body. In contrast with this stability of the unprotected biscrolled yarn BFC in human serum, providing 0.84 mW cm −2 (83%) after 24 h, and 0.77 mW cm −2 (76%) after 48 h ( Fig. 4b ) with continuous operation, previous unprotected BFCs working in human serum had low power output and short lifetimes [19] . Woven textile BFCs We exploited the mechanical robustness and flexibility of our biscrolled yarns to demonstrate one-compartment BFCs in which the anode and cathode yarn electrodes are either helically wound about a 1.2-mm diameter glass rod ( Fig. 5a ) or woven into a textile ( Fig. 5b ). The BFC textile was 5 mm wide and 7 mm long, and contained ~50-μm diameter anode and cathode yarns in the warp direction and 100-μm diameter polyester fibres in the weft direction. Four times as many cathode yarns as anode yarns were used to compensate for the lower cathodic current per yarn length. Total anode and cathode yarn lengths in each textile were 14 and 56 mm, respectively. A single textile BFC provided 128 μW maximum output power and an open-circuit voltage of 0.70 V ( Fig. 5c black symbols and curve). For two BFC textiles connected in series ( Fig. 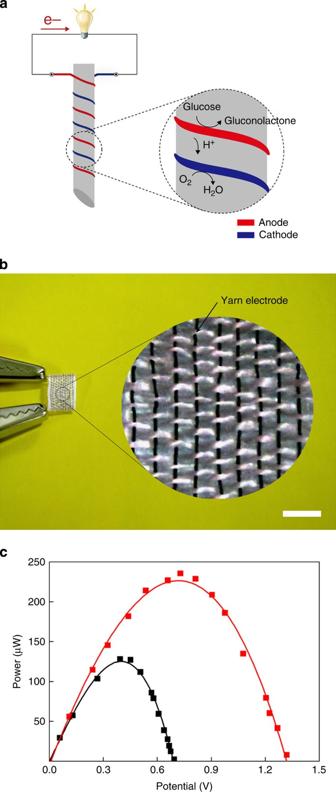Figure 5: Performance and structure for complete BFCs. (a) Schematic illustration of a biscrolled yarn BFC in which the anode and cathode are helically wrapped around a 1.2-mm diameter glass rod. (b) Photographs, at low and high magnifications, of a 5 mm by 7 mm woven textile BFC that deploys 50 μm diameter biscrolled yarn anodes and cathodes in the warp direction. Scale bar, 500 μm. (c) Power output as a function of potential for a woven textile BFC (black symbols and curve) and for two equivalent woven textile BFCs that are connected in series (red symbols and curve). 5c red symbols and curve), the maximum output power and the open-circuit voltage doubled to 229 μW and 1.32 V. Figure 5: Performance and structure for complete BFCs. ( a ) Schematic illustration of a biscrolled yarn BFC in which the anode and cathode are helically wrapped around a 1.2-mm diameter glass rod. ( b ) Photographs, at low and high magnifications, of a 5 mm by 7 mm woven textile BFC that deploys 50 μm diameter biscrolled yarn anodes and cathodes in the warp direction. Scale bar, 500 μm. ( c ) Power output as a function of potential for a woven textile BFC (black symbols and curve) and for two equivalent woven textile BFCs that are connected in series (red symbols and curve). Full size image This exceptional performance realized for the biscrolled yarn BFCs results in part from the yarn’s three-dimensional vascular structure. First of all, the corridors between scrolled PEDOT/MWCNT sheets in the biscrolled yarn provides a continuous internal pathway for rapid glucose and oxygen diffusion and ion transport from yarn surface to yarn center, as well as sufficient porosity through scroll layers for cross-layer transport ( Fig. 1 ; Supplementary Fig. 1 ). Hence, we have built upon previous BFC successes for yarns [3] , sheets [14] and disks [4] by providing a structure in which diffusion channels have distributed dimensions, like for the vascular system in the body. The hydrophilic PEDOT conducting polymer coating on the nanotubes not only enhances nanotube wettability, connectivity and conductivity, but also provides increased electrode stability in human serum. While electrolyte accessibility is provided within the entire yarn volume, incorporation of such anionic chemical species as urate, chloride and ascorbic acid from human serum is substantially avoided, which can decrease the performance of the anode [18] and cathode [17] . The improved stability in serum can be attributed to electrostatic interactions [20] that render the dopant anions relatively immobile in the conducting polymer. Hence, the PEDOT coating on the MWCNTs acts as a cation exchange membrane [21] . The PEDOT also facilitates high redox mediator and enzyme loadings from aqueous solution, contributes importantly to the yarn mechanical properties required for weaving ( Supplementary Fig. 2 ) and provides needed electronic conductivity. In addition, twist insertion in the PEDOT/MWCNT biscrolled yarn electrodes generates high compressive forces on the guest in yarn corridors, thereby effectively trapping this guest within the biscrolled yarn. These compressive forces provide intimate electronic contact for charge transfer between the biscrolled yarn guest and the yarn host current collector ( Fig. 1d,e ). Here, these mediated electron transfer-based systems usually have very efficient electron transfer between the enzyme and the electrode surface leading to larger current output [22] . However, the use of mediators in implantable devices could potentially generate issues with toxicity by the leakage of osmium or carbon nanotubes [23] . Similarly, stability of the device over its operating lifetime requires proper immobilization of the mediator and enzymes within the BFC. Several methods for the immobilization of polymers have increased the lifetime of enzymes by creating favourable microenvironments that allow for the facile diffusion of water and reactive species while protecting the electrode from degradation. Many approaches to increase stability also reduce electrical conductivity [24] . In our BFC system, however, coating of conductive polymer, PEDOT, can provide favourable microenvironments but also improve electrical conductivity of the electrodes. Further work is required to assess the long-term stability of these systems and investigate possible leakage of toxic agents. In conclusion, record high areal current densities for BFC anode and cathode, and record high volumetric power output based on total electrode volume were achieved using biscrolled carbon nanotube yarns. This performance as well as especially BFC stability in human serum and the weavability of the biscrolled yarn electrodes are encouraging for applications—perhaps even eventually for harvesting glucose chemical energy in the human body for powering implanted devices. Yarn guests The anodic enzyme was GOx from Aspergillus niger (219 U mg −1 ) purchased from Amano Enzyme Inc. (Japan). GOx was purified by using fast protein liquid chromatography on a cation exchange column [25] , [26] . The cathodic catalyst was BOD from Myrothecium verrucaria (10.5 U mg −1 , Sigma-Aldrich), which was used without purification. Poly(ethylene glycol) (400) diglycidyl ether (PEGDGE) from Polysciences Inc. was used as the cross-linker. The redox polymer mediators, (poly( N -vinylimidazole)-[Os(4,4′-dimethoxy-2,2′-bipyridine) 2 Cl]) +/2+ for the anode and (poly(acryl acid)-poly( N -vinylimidazole)-[Os(4,4′-dichloro-2,2′-bipyridine) 2 Cl]) +/2+ for the cathode, were synthesized using known methods [27] , [28] , [29] . All other chemicals used in this study were analytical reagent grade. Fabrication of enzyme-modified biscrolled yarn electrode MWCNT sheets were drawn from the sidewalls of MWCNT forests [8] and coated with vapour-phase polymerized PEDOT as previously reported [6] , [9] . Twist was inserted to obtain a yarn bias angle of ~40°, since use of higher twist angles degraded yarn strength and lower twist angles resulted in decreased areal current densities. The guest solutions for anodic and cathodic electrodes contained enzyme, redox mediator and cross-linker. The anodic catalyst consists of the cross-linked adduct of GOx (41 wt%), mediator I (52 wt%) and PEGDGE (7 wt%). The cathodic catalyst consists of BOD (41 wt%), mediator II (54 wt%) and PEGDGE (5 wt%). The optimal cross-linker concentration was determined on the basis of both output current density and stability of the BFC electrodes, as shown in the Supplementary Information ; ( supplementary Fig. 5 ) The maximum current density decreased and stability (for 6 h) increased with increasing cross-linker concentration. On the basis of this information, the cross-linker concentration was optimized for the cathode to maximize current output while maintaining high stability (>90%). For the anode electrode, a little higher wt% of the cross-linker than cathode was used owing to the critical consideration of stability based on the high current density (>20 mA cm −2 ). Redox mediator structures and electroactivity for anode (a, b) and cathode (c, d) are shown in supplementary Fig. 6 . Host PEDOT/MWCNT sheets containing 85 wt% PEDOT were immersed into either anodic and cathodic guest solutions, from which the guest materials were adsorbed on both sheet sides for 24 h at 4 °C. The host sheet was then twisted while still immersed in the guest solution using a low-speed motor, and the resulting biscrolled yarn electrode was finally cured for over 48 h at 4 °C. The total mass of each modified electrode for anode and cathode was determined before and after guest incorporation. The amount of immobilized guests was 25±1.3 μg for the anode electrode, and 13±0.5 μg for the cathode electrode. How to cite this article: Kwon, C. H. et al. High-power biofuel cell textiles from woven biscrolled carbon nanotube yarns. Nat. Commun. 5:3928 doi: 10.1038/ncomms4928 (2014).